Multimode circuit optomechanics near the quantum limit The coupling of distinct systems underlies nearly all physical phenomena. A basic instance is that of interacting harmonic oscillators, giving rise to, for example, the phonon eigenmodes in a lattice. Of particular importance are the interactions in hybrid quantum systems, which can combine the benefits of each part in quantum technologies. Here we investigate a hybrid optomechanical system having three degrees of freedom, consisting of a microwave cavity and two micromechanical beams with closely spaced frequencies around 32 MHz and no direct interaction. We record the first evidence of tripartite optomechanical mixing, implying that the eigenmodes are combinations of one photonic and two phononic modes. We identify an asymmetric dark mode having a long lifetime. Simultaneously, we operate the nearly macroscopic mechanical modes close to the motional quantum ground state, down to 1.8 thermal quanta, achieved by back-action cooling. These results constitute an important advance towards engineering of entangled motional states. One of the present goals in physics is the explanation of macroscopic phenomena as emerging from the quantum-mechanical laws governing nature on a microscopic scale. This understanding is also important for future quantum information applications [1] , [2] , [3] , [4] , as many of the most promising platforms are based on nearly macroscopic degrees of freedom. For macroscopic mechanical objects, their potential quantum behaviour [5] has been actively investigated with resonators interacting with an electromagnetic cavity mode [6] . In particular, freezing of the mechanical Brownian motion [7] , [8] down to below one quantum of energy has recently been observed [9] , [10] . Another result of radiation–pressure interaction is the mixing of the normal modes of vibration into linear combinations of the uncoupled phonon and photon modes. This has been verified with optomechanical Fabry–Perot cavity [11] , [12] , and by its on-chip microwave analogue [13] using an aluminium membrane. All this work is paving the way towards engineering non-classical motional [5] and hybrid quantum states [1] , [3] , [4] , [14] for basic tests of quantum theory [15] , [16] , as well as applications in foreseeable future. Corresponding phenomena in systems comprising more than two active degrees of freedom [17] , [18] , [19] have received less attention. In the optomechanical crystal set-up, coupling of mechanical vibrations via radiation–pressure interaction has been demonstrated with the zipper cavity [20] , however, with some direct interaction between the beams. In the microwave regime, such measurements have remained outstanding. In this work, we take a step further, and examine a multimode system where two micromechanical beams, having resonant frequencies ω 1 /(2 π )=32.1 MHz and ω 2 /(2 π )=32.5 MHz, are each coupled to a microwave on-chip cavity. We obtain the first evidence of hybridization of all the three degrees of freedom. This was made possible by operating, as opposed to the optical set-up, in the good-cavity limit, that is, both ω 1 and ω 2 were much larger than the cavity decay rate γ c . Simultaneously, the mechanical modes are found at low occupation numbers n m , near the quantum ground state, down to n m =1.8±0.5. These are the lowest occupations recorded with nanowire resonators to date, and they occur via the sideband cooling, starting from operation at dilution refrigerator temperatures at a few tens of millikelvin. Cavity with several mechanical modes In the optical domain [20] , a three-mode optomechanical system can be pictured as a Fabry–Perot cavity with both massive mirrors mounted via springs, see Fig. 1a . In the microwave version, ( Fig. 1b ), the mirrors are replaced by movable capacitors formed by the mechanical resonators. The electromechanical coupling arises when each mechanical resonator (labelled with j ), expressed as time-varying capacitors C j , independently modulates the total capacitance, and hence, the cavity frequency ω c . This is described by the coupling energies g j =( ω c /2 C ) ∂C j / ∂x j . In the actual device (see the micrograph in Fig. 1c ), the mechanical resonators are spatially separated by about 100 μm, and we hence expect the direct interaction between the beams via the substrate material to be negligible. We drive the cavity strongly by a microwave pump signal applied at the frequency ω P near the cavity frequency. The pump induces a large cavity field with the number of pump photons . This allows for a linearized description of the electromechanical interaction and results in substantially enhanced effective couplings , where is the zero-point amplitude. 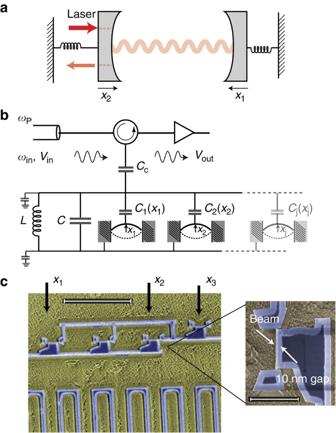Figure 1: Cavity-controlled coupling of micromechanical resonators. (a) Optomechanical system with both mirrors movable has three degrees of freedom. These are the optical field inside the Fabry–Perot cavity and the displacementsx1andx2of the mirrors. (b) Analogue of panelawith a microwave-regime cavity represented by the lumped element inductors and capacitors and arbitrary numberj=1 …Nof mechanical resonators. The system is probed through the coupling capacitorCcby shining a strong pump microwave tone (frequencyωP), which corresponds to the laser ina, and possibly a weak probe tone (frequencyωinand voltage amplitudeVin) in a dilution refrigerator down to 25 mK temperature. The outgoing waveVoutcan be monitored. (c) Images of the all-aluminium superconducting sample, showing four fabrication jigs for a beam. Total of three beams (x1…x3) were operating. Beams 1 and 2 had large electromechanical couplingsg1/2π=1.8 MHz nm−1,g2/2π=2.0 MHz nm−1, whereas the third beam had an order of magnitude smaller coupling. The scale bars are 50 μm on the left and 10 μm on the right. Figure 1: Cavity-controlled coupling of micromechanical resonators. ( a ) Optomechanical system with both mirrors movable has three degrees of freedom. These are the optical field inside the Fabry–Perot cavity and the displacements x 1 and x 2 of the mirrors. ( b ) Analogue of panel a with a microwave-regime cavity represented by the lumped element inductors and capacitors and arbitrary number j =1 … N of mechanical resonators. The system is probed through the coupling capacitor C c by shining a strong pump microwave tone (frequency ω P ), which corresponds to the laser in a , and possibly a weak probe tone (frequency ω in and voltage amplitude V in ) in a dilution refrigerator down to 25 mK temperature. The outgoing wave V out can be monitored. ( c ) Images of the all-aluminium superconducting sample, showing four fabrication jigs for a beam. Total of three beams ( x 1 … x 3 ) were operating. Beams 1 and 2 had large electromechanical couplings g 1 /2 π =1.8 MHz nm −1 , g 2 /2 π =2.0 MHz nm −1 , whereas the third beam had an order of magnitude smaller coupling. The scale bars are 50 μm on the left and 10 μm on the right. Full size image The general Hamiltonian for N mechanical resonators with frequencies ω j , individually coupled to a common cavity mode, written in a frame rotating with the pump, becomes Here, a is the annihilation operator for the cavity mode, while b j are those of the mechanical resonators. If one assumes roughly similar mechanical resonators, viz. and , the cavity becomes nearly resonant to all of them at the red-sideband detuned pump condition Δ=− ω m . Coupling of the mechanical resonators via the cavity ‘bus’ can be anticipated to be significant if the mechanical spectra begin to overlap when their width increased by the radiation pressure, γ eff = γ m + γ opt , grows comparable to the mechanical frequency spacing. Here, γ opt =4 G 2 / γ c . The equations of motion following from equation (1) allow one to verify the above assumption. We will in the following focus on two resonators, N =2. The result of such a calculation, which is detailed in the Supplementary Methods , is that they experience an effective coupling with energy G 12 = G 1 G 2 / γ c . In the limit of strong coupling, , the system is best described as a combination of two ‘bright’ modes with linewidths , and of a ‘dark’ mode having a long lifetime . In the latter, the two mechanical resonators oscillate out-of-phase and synchronize into a common frequency ( ω 1 + ω 2 )/2. In any case, the mode structure can be written with the normal coordinates for mode n , for position quadrature according to . Here we used the dimensionless amplitude of the mechanical oscillations , and similarly the dimensionless flux in the cavity. The mode expansion coefficients give the participation ratio of each uncoupled mode. They satisfy . In the experiment, we use doubly clamped flexural beams, which are made by the use of ion beam milling of aluminium [21] , having an ultranarrow nm vacuum slit to the opposite end of the cavity for maximizing the coupling. The cavity is a half-wavelength floating microstrip similar to the one used in Massel et al. [22] , resonating at ω c /(2 π )=6.98 GHz. The total cavity linewidth MHz is a sum of the internal damping γ I /(2 π )=1.4 MHz, and the external damping γ E /(2 π )=4.8 MHz. At the highest powers discussed, however, we obtain a decreased γ I /(2 π )=0.9 MHz, typical of dielectric loss mechanism. There are a total of three beams as shown in Fig. 1c . Two of the beams have a large zero-point coupling of g 1 x 01 /2 π =39 Hz and g 2 x 02 /2 π =44 Hz. The frequencies of beams 1 and 2 are relatively close to each other, kHz, such that it is straightforward to obtain an effective coupling G 12 of the same order. The third beam has an order of magnitude smaller coupling, and hence we neglect it in the full calculation, setting N =2 in equation (1) in what follows. The measurements are conducted in a cryogenic temperature below the superconducting transition temperature of the Al film ( K) to reduce losses. We used a dilution refrigerator set-up as in Massel et al. [22] down to 25 mK, which allows for a low mechanical mode temperature in equilibrium. Apart from this, cryogenic temperatures or superconductivity are not necessary [23] . Experimental data The modes can be probed by adding to the experimental set-up another, the probe, tone [11] , [13] , [22] with frequency ω in . The maximum pump power we can reach is 4 μW, inducing a coherent photon occupancy in the cavity, and effective coupling G 12 =(2 π ) × 150 kHz (with G 1 =0.93 MHz, G 2 =1.0 MHz). In Fig. 2a , we display changes of the cavity absorption by increasing the pump power. The two peaks at the bottom of the cavity dip are due to beams 1 and 2. They broaden with increasing n P , finally leaving behind a narrow dip between them. The overall lineshape is clearly not a sum of two Lorentzian peaks. 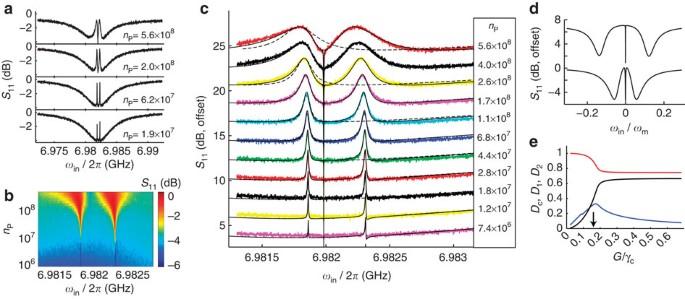Figure 2: Hybridization of microwave photons and two radio-frequency phonons. (a) Measured reflection coefficientS11=Vout/Vinof the probe microwave while a strong pump is applied at the red sideband,, at increasing pump amplitudes, from bottom to top. A low value ofS11means high resonance absorption. (b,c) Zoomed-in view of panela. An excellent agreement with the theory is obtained with reflection calculation using a complete model based on equation (1), for two beams 1 and 2 (solid lines). The dashed lines show a fit with an independent-resonator model for beam 1. The narrow feature at 6.982 GHz is due to beam 3. The curves are displaced vertically by 3 dB for clarity. (d) Theory plot for highernP; the dark mode is expected to become narrower and more and more phonon-like. Here, Δ=−(ω1+ω2)/2. The other parameter values areG/γc=0.28 and 0.63,nP=2 × 109and 1010, for the lower and upper curve, respectively. (e) Calculated dark mode decomposed into a linear combination of a photon and two phonons. Blue denotes the cavity componentDc, while red (D1) and black (D2) are components of the mechanical resonators 1 and 2, respectively. The parameters are as in panelc. The arrow denotes the highest experimental value. For simplicity, we takein panelsdande. Figure 2: Hybridization of microwave photons and two radio-frequency phonons. ( a ) Measured reflection coefficient S 11 = V out / V in of the probe microwave while a strong pump is applied at the red sideband, , at increasing pump amplitudes, from bottom to top. A low value of S 11 means high resonance absorption. ( b , c ) Zoomed-in view of panel a . An excellent agreement with the theory is obtained with reflection calculation using a complete model based on equation (1), for two beams 1 and 2 (solid lines). The dashed lines show a fit with an independent-resonator model for beam 1. The narrow feature at 6.982 GHz is due to beam 3. The curves are displaced vertically by 3 dB for clarity. ( d ) Theory plot for higher n P ; the dark mode is expected to become narrower and more and more phonon-like. Here, Δ=−( ω 1 + ω 2 )/2. The other parameter values are G / γ c =0.28 and 0.63, n P =2 × 10 9 and 10 10 , for the lower and upper curve, respectively. ( e ) Calculated dark mode decomposed into a linear combination of a photon and two phonons. Blue denotes the cavity component D c , while red ( D 1 ) and black ( D 2 ) are components of the mechanical resonators 1 and 2, respectively. The parameters are as in panel c . The arrow denotes the highest experimental value. For simplicity, we take in panels d and e . Full size image In Fig. 2c , we show a zoom-in view of the two peaks, together with theoretical predictions. One immediately sees that an attempt to simulate either peak by a single mechanical resonator coupled to cavity ( N =1 in the analysis), thereby neglecting the cavity-mediated coupling, fails to explain the lineshape at large . The full simulation with both beams 1 and 2 included, however, produces a remarkable agreement to the experiment. To create these curves, we further take into account a shift of the mechanical frequencies due to second-order interaction [8] , given as , where is the second-order coupling coefficient. The third beam, visible in Fig. 2c as a narrow feature just below 6.982 GHz, was later fitted by running a single-resonator calculation. This is justified because its mixing is negligible owing to weak coupling. The narrow dip between the peaks manifests the onset of the dark mode, where the cavity participation approaches zero with growing G j , as occurs also in other tripartite systems [24] . As usual for weakly decaying states, the dark modes can be useful for storage of quantum information [20] , [25] . The other two dips (best discerned in the theoretical plots at higher G j , see Fig. 2d ) are the bright modes, and they retain a fully mixed character of all three degrees of freedom. In Fig. 2e , we display the prediction for the mode expansion coefficients with respect to coupling. Asymmetry in the role of the mechanical modes is sensitive to parameters. With the maximum coupling in the experiment ( ), the normal modes are well mixed: the dark mode can be expressed as . One can also vary the pump detuning, thereby effectively detuning the cavity and the mechanical resonators [11] , [13] . An anticrossing of the cavity and mechanical modes is seen in Fig. 3a up to detuning , above which the system exhibits parametric oscillations. The pertinent simulation, Fig. 3b , portrays the main features of the measurement, except bending of the cavity frequency towards lower value in an upward sweep of Δ. We expect such possibly hysteretic behaviour of the cavity frequency to be due to second-order effects beyond the present linear model. 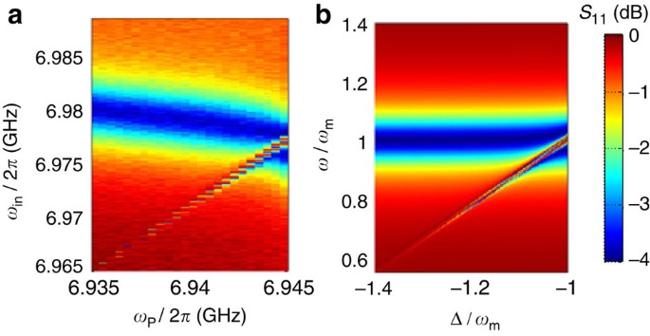Figure 3: Pump-detuning measurements. (a) Measured spectrum of the tripartite cavity electromechanical system when pumped at a fixed input power such that at resonance,,. The pump frequency was slowly swept from left to right. (b) Theory prediction. Figure 3: Pump-detuning measurements. ( a ) Measured spectrum of the tripartite cavity electromechanical system when pumped at a fixed input power such that at resonance, , . The pump frequency was slowly swept from left to right. ( b ) Theory prediction. Full size image Sideband cooling We now turn the discussion into showing how the tripartite system resides nearly in a pure quantum state during the mode-mixing experiments. The mechanical resonators can be sideband cooled with the radiation pressure back-action [8] , [26] , [27] , [28] under the effect of the pump, which also creates the mode mixing. Although the ground state of one mode was recently achieved this way [9] , [10] , cooling in multimode or nanowire systems is less advanced. The efficiency of cooling with two mechanical resonators is supposed to become hindered at those values of effective coupling where mode mixing starts to set in [29] . At modest pump powers, relevant for achieving the lowest phonon numbers in the present case, mixing remains insignificant. The incoherent output spectrum can be due to either a finite phonon number n m , or non-equilibrium population number of the cavity. The former manifests as a Lorentzian centred at the upper sideband, as in Fig. 4a , with the linewidth γ eff = γ m +4 G 2 / γ c , whereas the latter gives a small emission at broader bandwidth. The analytical approximation [8] and experimental details are discussed in Methods. 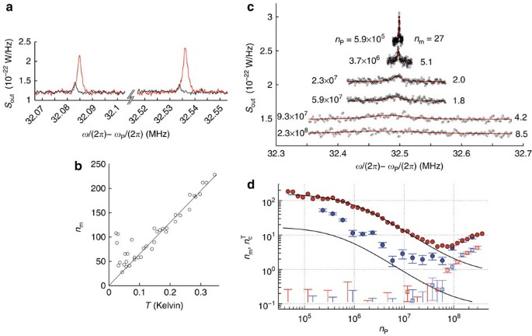Figure 4: Sideband cooling of motion down to 1.8 thermal quanta. (a) Cavity output spectra representing the thermal motion peaks of beams 1 (left) and 2 (right) measured at 345 mK (red) and 35 mK (black), withnP=4 × 105. (b) Calibration of the detection according to temperature dependence of the mechanical energy, given by the area of the peak (data for beam 2). The straight line is a linear fit to the data above 120 mK. (c) Output spectra of beam 2 at pump occupationnP, increasing from top to bottom. The curves are shifted vertically by 0.3y-axis units for clarity. The corresponding mechanical occupations are written on the right. (d) Progress of back-action cooling (beam 2) as a function of pump occupation. The mechanical mode temperature is given by circles, and the cavity temperature by squares. Red: high temperature, 245 mK; blue, base temperature (28 mK). The error bars are from the fits in panelc, given as one s.d. The ideal theoretical behaviour are plotted by the solid lines. Unless the data point for, including its error bars, was of positive sign, only the absolute value of the error bar is plotted. Figure 4: Sideband cooling of motion down to 1.8 thermal quanta. ( a ) Cavity output spectra representing the thermal motion peaks of beams 1 (left) and 2 (right) measured at 345 mK (red) and 35 mK (black), with n P =4 × 10 5 . ( b ) Calibration of the detection according to temperature dependence of the mechanical energy , given by the area of the peak (data for beam 2). The straight line is a linear fit to the data above 120 mK. ( c ) Output spectra of beam 2 at pump occupation n P , increasing from top to bottom. The curves are shifted vertically by 0.3 y -axis units for clarity. The corresponding mechanical occupations are written on the right. ( d ) Progress of back-action cooling (beam 2) as a function of pump occupation. The mechanical mode temperature is given by circles, and the cavity temperature by squares. Red: high temperature, 245 mK; blue, base temperature (28 mK). The error bars are from the fits in panel c , given as one s.d. The ideal theoretical behaviour are plotted by the solid lines. Unless the data point for , including its error bars, was of positive sign, only the absolute value of the error bar is plotted. Full size image At low input power, when the cavity back-action damping is small and , phonon number is set by thermal equipartition . This is best observed by the area of the mechanical peak in the output spectrum, as in Fig. 4a , which should be linear in cryostat temperature. The linearity holds down to about 150 mK temperatures ( Fig. 4b ), below which we observe intermittent heating, which is sensitive to parameters. The cooling of beam 2 is observed in the mechanical peaks shown in Fig. 4c (see Methods), and the resulting phonon numbers are displayed in Fig. 4d . At a relatively high temperature of 245 mK, the data points follow theory well up to input powers corresponding to . At the minimum cryostat temperature of 28 mK, the mode is not thermalized in a manner that depends irregularly on power. We obtain a minimum phonon number in beam 2 of , where the mechanical mode spends one-third of the time in the quantum ground state. The other mechanical mode, beam 1, cooled simultaneously down to 2.5 quanta, possibly compromised by the slightly smaller coupling. The cooling is quite clearly bottlenecked by heating, by the pump microwave, of the bath to which the mechanical mode is coupled. For the optimum data points, the starting temperature for cooling was raised to 150 mK, and above this it grows roughly quadratically with n P . The coupling of micromechanical resonators mediated via microwave photons in an on-chip cavity is a basic demonstration of the control of a multimode mechanical system near the quantum limit. The set-up provides a flexible platform for creation and studies of non-classical motional states entangled over the chip [30] , or over macroscopic distances [31] , [32] . The set-up is easily extended to embody nearly arbitrarily many mechanical resonators, hence allowing for designing an electromechanical metamaterial with microwave-tunable properties. For future quantum technology applications even at elevated temperatures [23] , data may be transferred for storage [33] from photonic modes into the dark states, which decay very slowly at the mechanical damping rate. Device fabrication The lithography to define the meandering cavity and jigs for the beams consisted of a single layer of electron-beam exposure, followed by evaporation of 150 nm of aluminium on a fused silica substrate. As the cavity is of planar structure, it has no potentially problematic cross-overs, which tend to have weak spots in superconducting properties and hence could heat up the cavity. We thus expect the cavity to portray a high critical current limited only by the intrinsic properties of the strip. With a 2 μm wide strip, we expect the critical current to be several milliamperes. With the maximum circulating currents in cavity ( Fig. 2 ), about 0.5 mA of the peak value, there was no sign of non-linearity in the cavity response. The mechanical resonators were defined by focussed ion beam cutting, as in Sulkko et al. [21] . We used low gallium ion currents of 1.5 pA, which gives the nominal beam width of about 7 nm. To maximize sputtering yield with minimal gallium contamination, we used a single-cutting pass mode. Otherwise, the cut beams tend to collapse to the gate. With the current recipe, fabrication of down to 10 nm gap widths over 5–10 μm distance can be done with about 50% yield. Theory of cavity-coupled resonators The Hamiltonian for N mechanical resonators each coupled to one cavity mode via the radiation–pressure interaction is The pump with the Hamiltonian induces a large cavity field with the number of pump photons . Under the strong driving, the cavity–mechanics interaction can be linearized individually for each beam, resulting in equation (1). Further details of the calculations are given in the Supplementary Methods . Sideband cooling For one beam, the measured output spectrum divided by system gain, S out ( ω ), carries information on the phonon number according to [8] which is a Lorentzian centred at the cavity frequency. A non-zero base level is due to possible broadband emission from the cavity, due to a thermal state with occupation . At modest pump (cooling) powers of utmost interest, coupling of the mechanical resonators remains insignificant, and thus we can apply equation (3) separately for each resonator. Some deviations can, however, occur at the highest powers with . To obtain the phonon number under strong back-action, we fit a Lorentzian to each peak as in Fig. 4c , obtaining independently the base level, amplitude and linewidth for every input power. These values are then compared with equation (3). This leaves, however, yet too many unknowns to obtain the occupations of the mechanics and cavity. This is basically because of uncertainties in the attenuations of both input and amplifier lines, which limit the accuracy of estimating n P . We can obtain a calibration using the linear temperature dependence, and by fitting the dependence of γ eff on input power. As opposed to, for instance, Rocheleau et al. [8] , the bottleneck for cooling is not heating of the cavity by strong pump, as seen in Fig. 4d , where the cavity temperature is increasing only little up to the optimum cooling powers corresponding to about 0.15 mA of peak current values in cavity. This can be due to the simplistic structure of the cavity. The above analysis supposes the presence of nearly no non-equilibrium photons in the cavity at zero or low input powers. This situation can be investigated by observing a possible emission from about cavity linewidth under these conditions. A complication arises because the cavity linewidth is so large that a small change is easily overwhelmed by modest standing waves in cabling. We avoided this issue by using temperature dependence of the cavity frequency, due to the kinetic inductance in the long microstrip. Thereby, a broad emission peak moving according to the cavity frequency would be easily distinguishable. We observed no such signal down to the level of , which justifies the above analysis. F.M. and T.H. developed the theory. J.-M.P., S.U.C. and M.A.S. contributed to design and fabrication of the samples, and cryogenic set-up. P.J.H. and M.A.S. conceived the work. How to cite this article: Massel, F. et al. Multimode circuit optomechanics near the quantum limit. Nat. Commun. 3:987 doi: 10.1038/ncomms1993 (2012).